Preotic neural crest cells contribute to coronary artery smooth muscle involving endothelin signalling Neural crest cells constitute a multipotent cell population that gives rise to diverse cell lineages. The neural crest arising from the postotic hindbrain is known as the ‘cardiac’ neural crest, and contributes to the great vessels and outflow tract endocardial cushions, but the neural crest contribution to structures within the heart remains largely controversial. Here we demonstrate that neural crest cells from the preotic region migrate into the heart and differentiate into coronary artery smooth muscle cells. Preotic neural crest cells preferentially distribute to the conotruncal region and interventricular septum. Ablation of the preotic neural crest causes abnormalities in coronary septal branch and orifice formation. Mice and chicks lacking endothelin signalling show similar abnormalities in the coronary artery, indicating its involvement in neural crest-dependent coronary artery formation. This is the first report that reveals the preotic neural crest contribution to heart development and smooth muscle heterogeneity within a coronary artery. The neural crest (NC), first identified by Wilhelm His in 1868 as ‘Zwischenstrang’, the intermediate cord [1] , is a multipotent stem cell population that originates from the border between the developing neural plate and surface ectoderm. NC cells (NCCs) can differentiate into a wide variety of cell types, including neurons, glia, pigment cells and craniofacial bones and cartilages in different developmental contexts [2] , [3] . In cardiovascular development, the cardiac NC arising from the postotic hindbrain corresponding to rhombomeres (r) 6–8 contributes to the formation of the tunica media of pharyngeal arch (PA) artery-derived great vessels, the aorticopulmonary septum and the outflow tract endocardial cushions [4] . Ablation of the cardiac NC in chick embryos results in aortic arch artery anomalies and persistent truncus arteriosus [5] , [6] , [7] . It has long been controversial whether and how the NC contributes to the formation of coronary arteries that supply the entire heart. Coronary arteries are generally accepted to form by ingrowth of angiogenic precursors into the aorta [8] , [9] , [10] , with the integration of migrating proepicardial mesenchyme as the main source of smooth muscle cells (SMCs) [11] , [12] , [13] . On the other hand, quail–chick chimera experiments have shown that the cardiac NC does not differentiate into coronary SMCs, although ganglia of NC origin are associated with the proximal portion of coronary arteries [10] , [14] . However, ablation of the cardiac NC results in disruption of the normal orifice formation and deployment of coronary arteries, indicating the role of NCCs in determining the spatial arrangement of the coronary vasculature [14] . By contrast, studies in mice have indicated the possible direct involvement of NCCs as the source of SMCs in the proximal coronary stems by using an NC-specific Wnt1 -Cre recombinase system [15] . The apparent discrepancy may be due to differences in species, but no definite explanation has been given for it. NC development involves multiple cell-to-cell interactions through a variety of signalling molecules. Endothelin-1 (Edn1), a 21-amino acid peptide known as the most potent vasoconstrictor [16] , is a key regulator of craniofacial and cardiovascular development, acting mainly on NCCs expressing Edn receptor type-A (Ednra), a G-protein-coupled receptor [17] , [18] , [19] . Inactivation of the Edn1–Ednra signalling leads to mandibular-to-maxillary homeotic-like transformation and cardiovascular anomalies, involving the outflow tract and aortic arch arteries [20] , [21] , [22] . In the present study, we newly identified anomalous coronary artery formation in Edn1 and Ednra knockout (KO) mice, which was associated with changes in the fate of NCCs. Furthermore, experiments in avian embryos first revealed that early-migrating preotic NCCs, rather than cardiac (postotic) NCCs, differentiate into SMCs and contribute directly to coronary artery formation partially through Edn1/Ednra-dependent mechanisms. Our findings may provide a solution to the controversy on the contribution of NCCs to coronary artery development. Coronary defects in the absence of Edn signalling During the analysis of cardiac phenotypes in Ednra KO mice, we often encountered abnormal structures in the interventricular septum. In E17.5 wild-type (WT) embryos, septal branches of the coronary artery were found along the right ventricular side of the interventricular septum ( Fig. 1a ). Ednra KO embryos instead showed large cavities in the septum ( Fig. 1d ). These cavities contained red blood cells and were lined by flat cells with endothelial morphology, indicating their vascular origin ( Fig. 1e ). In ventricular free walls, coronary arteries with apparently normal size were identified in both WT and Ednra KO mice ( Fig. 1c ). 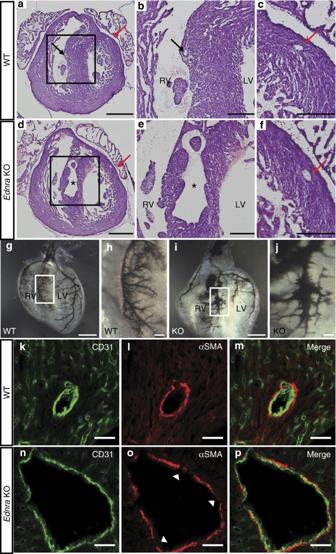Figure 1: Enlarged coronary artery branches inEdnraKO mice. (a–f) Haematoxylin-eosin staining of the frontal sections of WT (a–c) andEdnraKO(d–f) hearts. Boxed areas inaanddare magnified inbande, respectively.EdnraKO hearts exhibit enlarged vessels in the septum (asterisks) instead of the normal septal branches (black arrows). Areas around the left coronary arteries in the free wall (red arrows) are also magnified incandf, indicating no anatomical changes. (g–j) Coronary angiography by ink injection in WT (g,h) andEdnraKO (i,j) hearts. Boxed areas ingandiare magnified inhandj, respectively, indicating septal branch dilatation with an irregular and jagged contour. (k–p) Septal branch dilatation was diagnosed when its diameter was more than twice that of the proximal left coronary artery. Immunostaining of WT (k–m) andEdnraKO (n–p) septal branches for CD31 (k,n) and αSMA (l,o) with merged images (m,p). Smooth muscle layers are discontinuous in enlarged KO vessels (white arrowheads). All samples were collected at E17.5. RV, right ventricle; LV, left ventricle; scale bars, 500 (a,d,g,i), 200 (b,c,e,f), 100 (h,j) and 40 μm (k–p). Figure 1: Enlarged coronary artery branches in Ednra KO mice. ( a – f ) Haematoxylin-eosin staining of the frontal sections of WT ( a – c ) and Ednra KO( d – f ) hearts. Boxed areas in a and d are magnified in b and e , respectively. Ednra KO hearts exhibit enlarged vessels in the septum (asterisks) instead of the normal septal branches (black arrows). Areas around the left coronary arteries in the free wall (red arrows) are also magnified in c and f , indicating no anatomical changes. ( g – j ) Coronary angiography by ink injection in WT ( g , h ) and Ednra KO ( i , j ) hearts. Boxed areas in g and i are magnified in h and j , respectively, indicating septal branch dilatation with an irregular and jagged contour. ( k – p ) Septal branch dilatation was diagnosed when its diameter was more than twice that of the proximal left coronary artery. Immunostaining of WT ( k – m ) and Ednra KO ( n – p ) septal branches for CD31 ( k , n ) and αSMA ( l , o ) with merged images ( m , p ). Smooth muscle layers are discontinuous in enlarged KO vessels (white arrowheads). All samples were collected at E17.5. RV, right ventricle; LV, left ventricle; scale bars, 500 ( a , d , g , i ), 200 ( b , c , e , f ), 100 ( h , j ) and 40 μm ( k – p ). Full size image To characterize the nature of these abnormalities, we performed coronary angiography in E17.5 WT and KO embryos using an ink injection technique. This method revealed the branching structures of coronary arteries with a smooth contour and tapering toward the periphery in WT mice ( Fig. 1g ). By contrast, about 50% of Ednra KO embryos showed focal dilatation in the septal branch with a jagged contour ( Fig. 1i ). This phenotype was also found in Edn1 KO embryos with a similar penetrance ( Supplementary Fig. S1 ). Next we performed immunohistochemical analysis with anti-CD31 and anti-α-smooth muscle actin (αSMA) antibodies as markers for endothelial/endocardial cells and SMCs, respectively. In E17.5 WT mice, major coronary branches have a single and continuous smooth muscle layer surrounding an endothelial layer ( Fig. 1k–m ). In Ednra KO mice, however, enlarged septal branches partially lacked the SMC layer, although the endothelial layer appears intact ( Fig. 1n–p ), and a number of thin branches were sprouted from the enlarged vessels ( Fig. 1j ). These observations suggest that a disturbance in the formation of smooth muscle layer may cause the dilatation of coronary arteries in Ednra KO mice. Coronary angiography revealed another difference in coronary artery morphology between WT and Ednra - or Edn1 KO mice. In 90% of E17.5 WT mice on an Institute of Cancer Research (ICR) background, septal branches perfusing the interventricular septum originated from the right coronary artery ( Supplementary Fig. S2 and Supplementary Table S1 ). Serial observation during coronary formation indicated that this branching pattern was generated by remodelling, in which septal branches initially originating from the left coronary artery before E14.5 ( Fig. 2a and Supplementary Fig. S3 ) became connected to the right coronary artery through a communicating vessel around E15.5 ( Fig. 2b and Supplementary Fig. S3 ). This resulted in disappearance of the proximal part of the initial communication to the left coronary artery ( Supplementary Fig. S3 ). The communicating artery runs beneath the surface of the supraventricular crest and connects to the septal branch passing in the septomarginal trabeculation in adult mice ( Supplementary Fig. S3 ). In Edn1 KO mice, septal branches originated from the left coronary artery at E14.5 as in WT embryos ( Fig. 2e ). However, the communicating vessel to the right coronary artery did not form in Edn1 KO mice ( Fig. 2f ). Consequently, septal branches remained as branches from the left coronary artery in all the Edn1 KO mice examined ( Supplementary Table S1 ). Dilatation of the septal branch was also obvious at E15.5 ( Fig. 2f ). Ednra KO mice also exhibited the same phenotype ( Supplementary Table S1 ). In addition, the whole contour of coronary arteries, especially in the conotruncal region, was also affected in Edn1 - and Ednra KO mice ( Figs 1i and 2f and Supplementary Fig. S1 ), with dilatation of the proximal portion of the left coronary artery in some cases ( Supplementary Fig. S4 ). These results suggest that the Edn signalling may be critical for coronary artery development in mice. 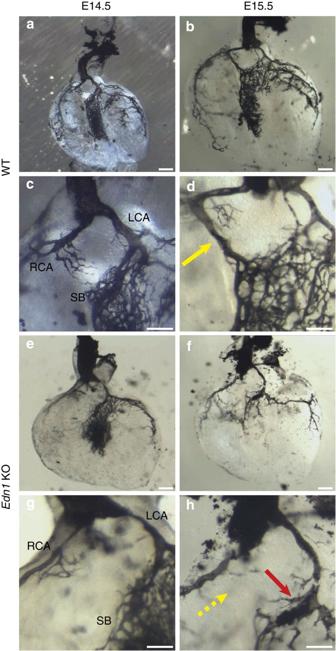Figure 2: Serial observation of septal branch formation. Coronary angiography by ink injection in WT (a–d) andEdn1KO (e–h) hearts at E14.5 (a,c,e,g) and E15.5 (b,d,f,h). The right-septal communicating artery is formed in the WT heart (d, yellow arrow), but not in theEdn1KO heart at E15.5 (h, yellow dotted arrow). The E15.5Edn1KO heart shows dilatation in the septal branch (red arrow). RCA, right coronary artery; LCA, left coronary artery; SB, septal branch; scale bars, 200 (a,b,e,f) and 100 μm (c,d,g,h). Figure 2: Serial observation of septal branch formation. Coronary angiography by ink injection in WT ( a – d ) and Edn1 KO ( e – h ) hearts at E14.5 ( a , c , e , g ) and E15.5 ( b , d , f , h ). The right-septal communicating artery is formed in the WT heart ( d , yellow arrow), but not in the Edn1 KO heart at E15.5 ( h , yellow dotted arrow). The E15.5 Edn1 KO heart shows dilatation in the septal branch (red arrow). RCA, right coronary artery; LCA, left coronary artery; SB, septal branch; scale bars, 200 ( a , b , e , f ) and 100 μm ( c , d , g , h ). Full size image As Edn1 KO mice show ventricular septal defect with about 50% penetrance [20] , it seemed possible that the coronary artery phenotype of the Edn1 - and Ednra KO mice might be secondary to ventricular septal defect (VSD). To test this possibility, we examined possible correlation between the incidence of VSD and coronary artery dilatation in serial sections of WT and Ednra KO mice. Among 19 KO mice on the ICR background, VSD and coronary dilatation were observed in 10 and 12 mice, respectively ( Supplementary Table S2 ). None of the 17 WT mice demonstrated such abnormalities ( Supplementary Table S2 and Supplementary Fig. S5 ). Notably, three mice showed VSD without coronary dilatation and, conversely, five mice showed coronary dilatation without VSD ( Supplementary Table S2 and Supplementary Fig. S5 ). This result suggests that VSD and coronary dilatation are independent of each other in Ednra KO mice. Wnt1-Cre -labelled cells contribute to coronary smooth muscle To test whether the coronary artery abnormalities are due to NC defects, we used Wnt1-Cre /R26R reporter mice that express β-galactosidase from the ROSA26 locus upon Cre-mediated recombination. Although the contribution of Wnt1-Cre -labelled cells to the walls of proximal coronary arteries has been previously reported [15] , their distribution patterns and ultimate cell types remain elusive. Therefore, we first analysed the temporal and spatial distribution of Wnt1-Cre -labelled cells along the coronary vasculature. At E13.5, Wnt1-Cre -labelled cells were found in the conotruncal region to form the condensed mesenchyme as previously reported for NCCs [7] , [15] , and also around the proximal coronary vessels, although they did not express contractile marker proteins ( Supplementary Fig. S6 ). At E14.5, the expression of αSMA was detected in labelled cells around the proximal coronary arteries ( Supplementary Fig. S6 ). Labelled cells were also detected around more distal vessels in the interventricular septum, but they did not express αSMA ( Supplementary Fig. S6 ). At E17.5, labelled cells were found to converge on the proximal portion of coronary arteries ( Fig. 3a–c ). Immunohistochemical analysis revealed that these labelled cells were incorporated into the αSMA-positive smooth muscle layer together with Wnt1-Cre -negative cells, whereas many Wnt1-Cre -labelled cells outside the smooth muscle layer remained αSMA-negative ( Fig. 3d–f ). We could not find Wnt1-Cre -labelled cells in any coronary branches in the apical region. At intermediate locations, however, labelled cells were observed in the septal branch ( Fig. 3g–i ) contributing directly to the αSMA-positive SMCs ( Fig. 3j–l ). 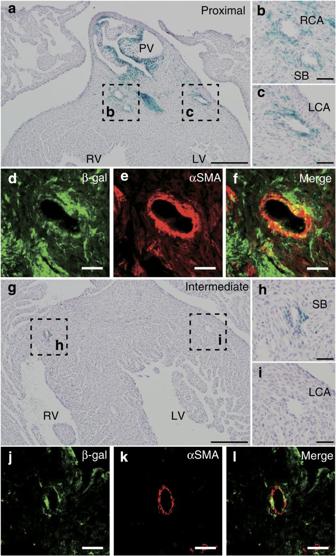Figure 3: Spatial patterns ofWnt1-Cre-labelled cells. Frontal sections of hearts from E17.5Wnt1-Cre/R26R mice at proximal (a–f) and intermediate (g–l) level.Wnt1-Cre-labelled cells are detected by staining for β-galactosidase (β-gal) enzyme activity (a–c,g–i) and immunoreactivity (d–f,j–l). Boxed areas inaandgare magnified inbandc, andhandi, respectively.Wnt1-Cre-labelled cells converge on the proximal coronary arteries (b,c) and septal branches (h). Co-immunostaining for β-gal and αSMA shows their smooth muscle phenotype in the proximal coronary arteries (d–f) and septal branches (j–l). PV, pulmonary valve; RCA, right coronary artery; LCA, left coronary artery; RV, right ventricle; LV, left ventricle; SB, septal branch; scale bars, 200 (a,g) and 40 μm (d–f,j–l). Figure 3: Spatial patterns of Wnt1-Cre -labelled cells. Frontal sections of hearts from E17.5 Wnt1-Cre /R26R mice at proximal ( a – f ) and intermediate ( g – l ) level. Wnt1-Cre -labelled cells are detected by staining for β-galactosidase (β-gal) enzyme activity ( a – c , g – i ) and immunoreactivity ( d – f , j – l ). Boxed areas in a and g are magnified in b and c , and h and i , respectively. Wnt1-Cre -labelled cells converge on the proximal coronary arteries ( b , c ) and septal branches ( h ). Co-immunostaining for β-gal and αSMA shows their smooth muscle phenotype in the proximal coronary arteries ( d – f ) and septal branches ( j – l ). PV, pulmonary valve; RCA, right coronary artery; LCA, left coronary artery; RV, right ventricle; LV, left ventricle; SB, septal branch; scale bars, 200 ( a , g ) and 40 μm ( d – f , j – l ). Full size image Next we analysed the distribution of Wnt1-Cre -labelled cells in Ednra KO embryos. At E13.5–E14.5, Wnt1-Cre -labelled cells were abundantly found in the conotruncal region and formed the condensed mesenchyme in KO embryos as seen in WT and heterozygous embryos ( Supplementary Fig. S6, S7 ). However, they were not detected around the proximal coronary arteries in KO embryos ( Supplementary Fig. S7 ), unlike in WT embryos ( Supplementary Fig. S6 ). Also at E17.5, no labelled cells were found around the enlarged septal branch in KO embryos, whereas a number of labelled cells were observed around the septal branch in heterozygous embryos ( Fig. 4a–d ). Consequently, the abnormal septal branch in KO embryos lacked Wnt1-Cre -labelled SMCs, which were constantly observed in the septal branch of heterozygous embryos ( Fig. 4e–j ). Even in the proximal region, Wnt1-Cre -labelled cells, although appearing in the vicinity of the vessel wall, were hardly detectable in the smooth muscle layer in Ednra KO embryos, whereas heterozygous littermates showed incorporation of labelled cells into the smooth muscle layer as observed in WT embryos ( Fig. 4k-p ). By contrast, labelled cells were abundantly incorporated into the tunica media of the aorta and had differentiated into SMCs in Ednra KO embryos, as well as in heterozygous or WT littermates ( Supplementary Figs S8 and S9 ), indicating that the contribution of Wnt1-Cre -labelled cells to the wall of the aorta and coronary arteries are differentially regulated in terms of their requirement for Edn signalling. 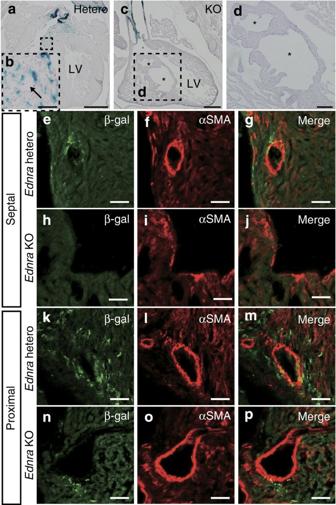Figure 4: Lack ofWnt1-Cre-labelled SMCs in the coronary artery ofEdnraKO mice. Frontal sections of hearts fromWnt1-Cre/R26R mice withEdnraEGFP/+heterozygous (Hetero) (a,b,e–g,k–m) orEdnraEGFP/EGFPhomozygous (KO;c,d,h–j,n–p) alleles.Wnt1-Cre-labelled cells are detected by staining for β-galactosidase (β-gal) activity (a–d) and immunoreactivity (e–p). Septal branches boxed inaandcare magnified inb(black arrow) andd(asterisks), respectively. Few labelled cells are detected in the dilated septal branch of KO hearts. Co-immunostaining for β-gal (e,h,k,n) and αSMA (f,i,l,o) with merged images (g,j,m,p) shows decreases inWnt1-Cre-labelled SMCs in the septal branch (e,h) and in the proximal artery (k,n). LV, left ventricle; scale bars, 500 (a,c) and 40 μm in (b,d,e–p). Figure 4: Lack of Wnt1-Cre -labelled SMCs in the coronary artery of Ednra KO mice. Frontal sections of hearts from Wnt1-Cre /R26R mice with Ednra EGFP/+ heterozygous (Hetero) ( a , b , e – g , k – m ) or Ednra EGFP/EGFP homozygous (KO; c , d , h – j , n – p ) alleles. Wnt1-Cre -labelled cells are detected by staining for β-galactosidase (β-gal) activity ( a – d ) and immunoreactivity ( e – p ). Septal branches boxed in a and c are magnified in b (black arrow) and d (asterisks), respectively. Few labelled cells are detected in the dilated septal branch of KO hearts. Co-immunostaining for β-gal ( e , h , k , n ) and αSMA ( f , i , l , o ) with merged images ( g , j , m , p ) shows decreases in Wnt1-Cre -labelled SMCs in the septal branch ( e , h ) and in the proximal artery ( k , n ). LV, left ventricle; scale bars, 500 ( a , c ) and 40 μm in ( b , d , e – p ). Full size image Edn1 and Ednra expression in mouse developing heart To investigate the involvement of Edn signalling in coronary development, we examined Edn1 and Ednra expression in developing heart. At E12.5, when primary coronary vascular plexus starts to form [23] , Edn1 was expressed in the outflow and atrioventricular cushion endocardium and developing interventricular septum ( Fig. 5a and Supplementary Fig. S10 ). At E13.5–E14.5, Edn1 expression appeared in the endothelium of the proximal portions of coronary arteries in addition to the cushion and septal endocardium ( Fig. 5b and Supplementary Fig. S10 ). Ednra expression, mimicked by knocked-in EGFP expression [18] , [24] , was detected broadly in cardiomyocytes and aortic SMCs, and also in Wnt1-Cre -labelled cells in the condensed mesenchyme and close to the endocardium at E12.5 ( Fig. 5d–f ). This region is likely to be the site where the communicating artery between the right coronary artery and the septal branch is forming ( Supplementary Fig. S3 ). At E13.5 and E14.5, Ednra-EGFP was expressed in Wnt1-Cre -labelled cells in condensed mesenchyme and around coronary arteries ( Fig. 5g–l ). These results indicate that Edn1 secreted from the cushion endocardium and later from the coronary endothelium may recruit Wnt1-Cre -labelled cells by acting on Ednra, and promote their differentiation into coronary artery SMCs. 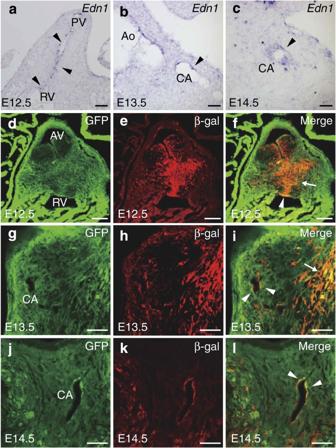Figure 5: Distribution patterns ofEdn1expression andEdnra-EGFP-positiveWnt1-Cre-labelled cells. (a–c)In situhybridization forEdn1in WT hearts. At E12.5 (a),Edn1expression is detected in the conotruncal cushion endocardium (arrowheads). At E13.5 (b) and E14.5 (c), the endothelium of proximal coronary arteries in the conal region expressesEdn1(arrowheads). (d–l) Co-immunostaining for enhanced green fluorescent protein (EGFP) and β-galactosidase (β-gal) in the hearts ofWnt1-Cre/R26R; EdnraEGFP/+mice. EGFP expression is driven by the endogenousEdnrapromoter and reflectsEdnraexpression. At E12.5, EGFP signals were detected broadly in cardiomyocytes and aortic SMCs, and also inWnt1-Cre-labelled cells in the condensed mesenchyme (arrow) and close to the endocardium (arrowhead;d–f). At E13.5 and E14.5, EGFP was expressed inWnt1-Cre-labelled cells in the condensed mesenchyme (arrow) around coronary arteries (arrowheads;g–i,j–l). Ao, aorta; CA, coronary artery; PV, pulmonary valve primordium; RV, right ventricle; scale bars, 100 (d–f) and 40 μm (a–c,g–l). Figure 5: Distribution patterns of Edn1 expression and Ednra-EGFP -positive Wnt1-Cre -labelled cells. ( a – c ) In situ hybridization for Edn1 in WT hearts. At E12.5 ( a ), Edn1 expression is detected in the conotruncal cushion endocardium (arrowheads). At E13.5 ( b ) and E14.5 ( c ), the endothelium of proximal coronary arteries in the conal region expresses Edn1 (arrowheads). ( d – l ) Co-immunostaining for enhanced green fluorescent protein (EGFP) and β-galactosidase (β-gal) in the hearts of Wnt1-Cre/ R26R ; Ednra EGFP/+ mice. EGFP expression is driven by the endogenous Ednra promoter and reflects Ednra expression. At E12.5, EGFP signals were detected broadly in cardiomyocytes and aortic SMCs, and also in Wnt1-Cre -labelled cells in the condensed mesenchyme (arrow) and close to the endocardium (arrowhead; d – f ). At E13.5 and E14.5, EGFP was expressed in Wnt1-Cre -labelled cells in the condensed mesenchyme (arrow) around coronary arteries (arrowheads; g – i , j – l ). Ao, aorta; CA, coronary artery; PV, pulmonary valve primordium; RV, right ventricle; scale bars, 100 ( d – f ) and 40 μm ( a – c , g – l ). Full size image Preotic NCCs contribute to coronary artery smooth muscle To assure that Wnt1-Cre -labelled cells contributing to the coronary artery represented NC derivatives, we used the quail–chick chimera technique for accurate lineage tracing. However, chimeric replacement of the postotic NC at the level of r6–r8 in chick embryos followed by staining with a quail-specific QCPN antibody showed no contribution of quail cells to the wall of coronary arteries, although some were detected within the conotruncal and septal region ( Supplementary Fig. S11 and Supplementary Movie S1 ). We then hypothesized that more anterior NCCs might contribute to the coronary arteries and generated quail–chick chimeras in which the midbrain and preotic hindbrain (r1–r5) neural folds were bilaterally excised and replaced by orthotopic quail grafts at 3–7 somite stages (ss; Fig. 6a ). Surprisingly, replacement of the preotic NC resulted in a significant number of QCPN-positive quail cells distributing into the heart, especially in the interventricular septum ( Fig. 6b–d ). Quite a few QCPN-positive cells were found to be incorporated into the smooth muscle layer of the coronary arteries in a pattern similar to that of Wnt1-Cre -labelled cells in mouse embryos ( Fig. 6b ), whereas many other QCPN-positive cells were scattered within cardiac tissues, especially in papillary muscles in the right ventricle ( Fig. 6c ). Co-immunostaining for desmin, a marker for cardiomyocytes, indicated that QCPN-positive cells within the cardiac tissue represented a non-cardiomyocyte population ( Supplementary Fig. S12 ). 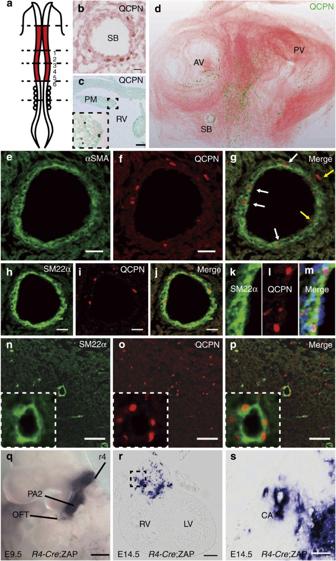Figure 6: Quail–chick chimeras reveal the contribution of preotic NCCs to developing coronary arteries. (a) Scheme illustrating the position of the preotic NC grafted. The quail preotic NC between the midbrain and r5 was orthotopically grafted to chick embryos. (b,c) QCPN immunostaining for quail nuclei, indicating QCPN-positive cells in the septal branch (b) and papillary muscles in the right ventricle (c). QCPN-positive cells in the papillary muscle are magnified in the left lower inset (c). (d) Three-dimensional reconstruction of immunostained sections. One hundred and twenty horizontal sections of 4 μm each were used for the reconstruction. QCPN-labelled cells distribute mainly to the interventricular septum and the septal branch. (e–m) Immunohistochemistry in the septal branch with antibodies to αSMA (e) or SM22α (h,n) and QCPN (f,i,o), with merged images (g,j,p) shows the contribution of QCPN-labelled cells to SMCs (white arrows) and possibly non-muscle cells (yellow arrows). Magnified images ofjreveal that QCPN-labelled nuclei are visible in the tunica media (k–m). (n–p) Immunohistochemistry in a small branch of the coronary artery with antibodies to SM22α (n) and QCPN (o), with merged images (p). Magnified images are shown in the left lower insets. (q–s)R4-Cre-labelled cells are detected by alkaline phosphatase staining. At E9.5,R4-Cre-labelled cells are specifically expressed in PA2 and the outflow tract (q). At E14.5, section staining shows their expression in the conal region (r). Boxed area inris magnified ins, a coronary artery is covered withR4-Cre-labelled cells. AV, aortic valve; PV, pulmonary valve; CA, coronary artery; OFT, outflow tract; PA2, second pharyngeal arch; PM, papillary muscle; RV, right ventricle; LV, left ventricle; SB, septal branch; scale bars, 500 (q), 200 (r), 100 (c), 10 (b) and 40 μm (e–j,n–p). Figure 6: Quail–chick chimeras reveal the contribution of preotic NCCs to developing coronary arteries. ( a ) Scheme illustrating the position of the preotic NC grafted. The quail preotic NC between the midbrain and r5 was orthotopically grafted to chick embryos. ( b , c ) QCPN immunostaining for quail nuclei, indicating QCPN-positive cells in the septal branch ( b ) and papillary muscles in the right ventricle ( c ). QCPN-positive cells in the papillary muscle are magnified in the left lower inset ( c ). ( d ) Three-dimensional reconstruction of immunostained sections. One hundred and twenty horizontal sections of 4 μm each were used for the reconstruction. QCPN-labelled cells distribute mainly to the interventricular septum and the septal branch. ( e – m ) Immunohistochemistry in the septal branch with antibodies to αSMA ( e ) or SM22α ( h , n ) and QCPN ( f , i , o ), with merged images ( g , j , p ) shows the contribution of QCPN-labelled cells to SMCs (white arrows) and possibly non-muscle cells (yellow arrows). Magnified images of j reveal that QCPN-labelled nuclei are visible in the tunica media ( k – m ). ( n – p ) Immunohistochemistry in a small branch of the coronary artery with antibodies to SM22α ( n ) and QCPN ( o ), with merged images ( p ). Magnified images are shown in the left lower insets. ( q – s ) R4-Cre -labelled cells are detected by alkaline phosphatase staining. At E9.5, R4-Cre -labelled cells are specifically expressed in PA2 and the outflow tract ( q ). At E14.5, section staining shows their expression in the conal region ( r ). Boxed area in r is magnified in s , a coronary artery is covered with R4-Cre -labelled cells. AV, aortic valve; PV, pulmonary valve; CA, coronary artery; OFT, outflow tract; PA2, second pharyngeal arch; PM, papillary muscle; RV, right ventricle; LV, left ventricle; SB, septal branch; scale bars, 500 ( q ), 200 ( r ), 100 ( c ), 10 ( b ) and 40 μm ( e – j , n – p ). Full size image To obtain the whole pattern of their distribution, we reconstructed the sections staining and plotted QCPN-positive cells ( Fig. 6d ). They showed a unique pattern of distribution, that is, quail cells were abundant in the upper part of the interventricular septum ( Fig. 6d and Supplementary Movie S2 ). Immunohistochemical analysis revealed that these quail cells contributed to SMCs and possibly non-muscle cells ( Fig. 6e–g ). SM22α, another smooth muscle marker, was expressed in QCPN-positive cells in the septal branch ( Fig. 6h–m ) In small vessels around the conotruncal region, QCPN- and SM22α-positive SMCs were abundantly found ( Fig. 6n–p ). Orthotopic grafting of quail proepicardial tissues into chick embryos revealed that QCPN-negative SMCs in the septal branch, as well as in arteries in the free wall, are predominantly of proepicardial origin ( Supplementary Fig. S13 ), as reported previously [11] , [12] , [13] . Then we subdivided the grafted region of the preotic NC ( Supplementary Fig. S14 ) and found that all regions of the preotic NCCs contributed to papillary muscles. However, we found no contribution of NCCs originating from the midbrain to r2 in the septal branch or upper part of the interventricular septum, showing that the cells that originated from r3 to r5 might mainly contribute to coronary artery smooth muscle. As both r3 and r5 provide only a small population of migratory NCCs [25] , we examined whether r4 is responsible for NC contribution to coronary artery smooth muscle by using R4::Cre;Z/AP transgenic mouse embryos, in which r4-derived NCCs were specifically and permanently labelled by alkaline phosphatase (AP) expression. At E9.5, AP-positive cells were detected in the outflow tract in addition to the second PA (PA2; Fig. 6q ). At E11.5, AP-positive cells were found in PA2 mesenchyme and cardiac outflow cushion tissue, but not in the third to sixth pharyngeal arteries contributed by postotic NCCs ( Supplementary Fig. S15 ). At E14.5, AP-positive cells were detected in the conotruncal region and formed a layer surrounding proximal coronary arteries in addition to their contribution to PA2-derived ear structures ( Fig. 6r and Supplementary Fig. S15 ). These results indicate that the contribution of preotic NCCs to cardiovascular development is distinct from that of postotic NCCs, and that NCCs from r4 mainly contribute to coronary artery SMCs. Finally, we examined spatiotemporal relationship between preotic and postotic NCCs by labelling premigratory crest cells with fluorescent dyes. We injected CM-DiI (red) and CFDA/DiO (green) into the neural folds at the levels of r3/4 (preotic) and somites 1/2 (postotic) in chick embryos at 8 ss and examined fluorescent signals after 3 days of incubation ( Fig. 7a ). Interestingly, migration of preotic crest cells preceded that of postotic cells in the similar pathway within the cushion tissue ( Fig. 7b–d ), indicating that the anteroposterior order of NCCs corresponds to their proximodistal location within the cardiac region through different timing of migration. 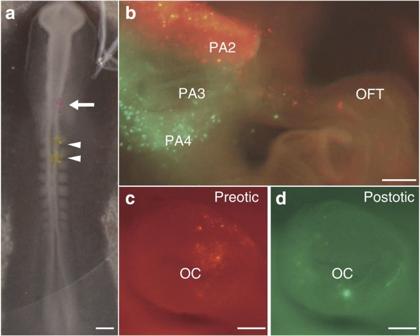Figure 7: Dual labelling of both preotic and postotic NCCs. (a,b) CM-DiI (red) and CFDA/DiO (green) were simultaneously injected into the neural fold at the levels of r3/4 (preotic, arrow) and somite 1/2 (postotic, arrowheads), respectively (a). At day3, each dye marks migratory cells in their corresponding PAs and the outflow tract (OFT). Migration of CM-DiI-labelled preotic crest cells preceded that of CFDA-DiO-labelled postotic cells (b). (c,d) Sections of the OFT reveal each dye troops through outflow cushions. OC, outflow cushion; PA2–4, the second to fourth PAs; scale bars, 200 μm (b). Figure 7: Dual labelling of both preotic and postotic NCCs. ( a , b ) CM-DiI (red) and CFDA/DiO (green) were simultaneously injected into the neural fold at the levels of r3/4 (preotic, arrow) and somite 1/2 (postotic, arrowheads), respectively ( a ). At day3, each dye marks migratory cells in their corresponding PAs and the outflow tract (OFT). Migration of CM-DiI-labelled preotic crest cells preceded that of CFDA-DiO-labelled postotic cells ( b ). ( c , d ) Sections of the OFT reveal each dye troops through outflow cushions. OC, outflow cushion; PA2–4, the second to fourth PAs; scale bars, 200 μm ( b ). Full size image Preotic NC ablation causes coronary artery malformations Next we ablated the preotic NC from the midbrain to r5 and analysed the coronary morphology after 12 days of incubation to examine its role in coronary development. Unlike in postotic NC-ablated embryos, no great vessel anomalies were observed in preotic NC-ablated embryos ( Fig. 8a ). Instead, coronary artery malformations were detected in about one-third of ablated embryos ( Supplementary Table S3 ). Some preotic NC-ablated embryos showed extra ostium formation even in the non-coronary cusp, where the extra ostium is never formed in normal embryos ( Fig. 8c ). Coronary angiography also revealed abnormally enlarged septal branches like those of Edn1-/Ednra KO mice ( Fig. 8e ). To avoid any artificial effect caused by intravascular injection, we also generated reconstructed serial sections for three-dimensional analysis. Angiography, stained sections and reconstructed images all showed dilated septal branches ( Fig. 8g ), and reconstitution image recaptured the same finding of the coronary angiography ( Fig. 8i–l ). Furthermore, we also found a fistula between the septal branch and the right ventricle or other types of anomalies, including septal branch split into two lumens or more by a pillar-like structure in ablated embryos ( Fig. 8k and Supplementary Fig. S16 ). The enlarged septal branch partially lacked the marker of SMCs ( Fig. 8m ). These deformities might reflect abnormalities in the remodelling process. 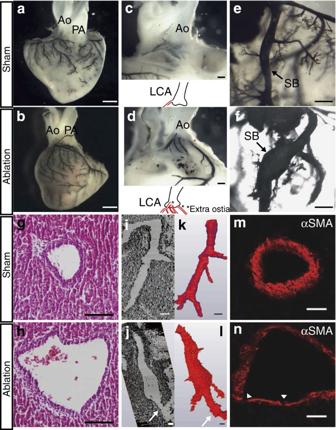Figure 8: Preotic NC ablation leads to coronary artery malformations. (a–f) Coronary angiography in sham-operated (a,c,e) and NC-ablated (b,d,f) embryos. Whereas the ablated embryos show no apparent great vessel abnormalities (b), they demonstrate superfluous coronary ostia (d) and enlarged septal branches (f). (g–l) Haematoxylin-eosin staining (g,h) with two-dimensional (i,j) and three-dimensional (k,l) reconstructions in sham-operated (g,i,k) and NC-ablated (h,j,l) embryos shows an enlarged septal branch with an irregular contour and the fistula to the right ventricle (white arrows) in the ablated embryo (j,l). One hundred and ninety horizontal sections of 10 μm each were used for the reconstruction. (m,n) Immunohistochemistry in the septal branch with antibodies to αSMA in sham-operated (m) and NC-ablated (n) embryos. The ablated embryo shows a discontinuous smooth muscle layer in the septal branch (white arrowheads). Ao, Aorta; LCA, left coronary artery; PA, pulmonary artery; SB, septal branch; scale bars, 1 mm (a,b), 200 (e,f),100 (c,d) and 40 μm (g,h,m,n), and 100 arbitrary units (a.u.;i–l). Figure 8: Preotic NC ablation leads to coronary artery malformations. ( a – f ) Coronary angiography in sham-operated ( a , c , e ) and NC-ablated ( b , d , f ) embryos. Whereas the ablated embryos show no apparent great vessel abnormalities ( b ), they demonstrate superfluous coronary ostia ( d ) and enlarged septal branches ( f ). ( g – l ) Haematoxylin-eosin staining ( g , h ) with two-dimensional ( i , j ) and three-dimensional ( k , l ) reconstructions in sham-operated ( g , i , k ) and NC-ablated ( h , j , l ) embryos shows an enlarged septal branch with an irregular contour and the fistula to the right ventricle (white arrows) in the ablated embryo ( j , l ). One hundred and ninety horizontal sections of 10 μm each were used for the reconstruction. ( m , n ) Immunohistochemistry in the septal branch with antibodies to αSMA in sham-operated ( m ) and NC-ablated ( n ) embryos. The ablated embryo shows a discontinuous smooth muscle layer in the septal branch (white arrowheads). Ao, Aorta; LCA, left coronary artery; PA, pulmonary artery; SB, septal branch; scale bars, 1 mm ( a , b ), 200 ( e , f ),100 ( c , d ) and 40 μm ( g , h , m , n ), and 100 arbitrary units (a.u. ; i – l ). Full size image We also performed a region-specific preotic NC ablation before 7 ss, and most frequently found septal branch malformations when the NC between r3 to r5 was ablated ( Supplementary Table S3 ). No abnormalities appeared when the ablation was performed at later stages ( Supplementary Table S3 ). Considering that cardiac (postotic) NC ablations are routinely performed after 7 ss, our findings are consistent with the earlier migration of preotic NCCs than postotic cardiac NCCs. Finally, we examined whether inactivation of Edn signalling can cause coronary artery abnormalities also in chick embryos using bosentan, an Edn receptor antagonist. Bosentan-treated embryos displayed enlarged septal branches as in Edn1 and Ednra KO mice and preotic NC-ablated chick embryos ( Supplementary Fig. S17 ). This result suggests that Edn signalling is involved in the contribution of NCCs to coronary artery formation in both mouse and chick embryos. The regional destination and cell fate of NCCs correspond to their premigratory position within the neural tube along the anteroposterior axis [2] . The contribution of NCCs to cardiac development has been attributed uniquely to those arising from the postotic hindbrain, referred to as the cardiac NC [4] . In this study, we first identified the contribution of the preotic cranial NC, which primarily gives rise to the craniofacial skeleton [3] , to developing coronary arteries and adjacent cardiac tissues ( Supplementary Fig. S18 ). This study has also reconciled the long-lasting controversy on the contribution of NCCs to coronary artery development, and has shown that the discrepancy between mouse and chick/quail experiments is not due to a species difference. The distribution pattern of preotic NCCs and their contribution to cardiovascular development are obviously different from those of the postotic cardiac NC. Although cardiac NCCs arising from the postotic hindbrain migrate into the posterior (caudal) PAs and form the tunica media of PA artery-derived great vessels, the aorticopulmonary septum and the outflow tract endocardial cushions, preotic NCCs migrate into the heart beyond the conotruncal region and give rise to coronary SMCs and mesenchymal-like cells, especially in the interventricular septum and papillary muscles of the right ventricle. This fate is limited to the NCCs that migrate very early from the neural folds of the midbrain and preotic (r1–r5) hindbrain, which may explain why this cell population has hitherto escaped detection. Together with dual labelling experiments, the spatiotemporal order of NCCs along the anteroposterior axis appears to correspond to their postmigratory positions within the cardiovascular system along the inflow–outflow axis. Ablation of the postotic and preotic NC in chick embryos leads to different types of coronary artery defects, indicating their roles in coronary artery development through different mechanisms. In the absence of postotic NCCs, the coronary arteries show a variance in their site of origin and an asymmetry in the deployment of SMCs [14] . However, concomitant persistent truncus arteriosus with changes in NC-related structures, such as the myocardial sheath, and no direct contribution of postotic NCCs to the coronary smooth muscle make the direct involvement of the postotic NC obscure. By contrast, ablation of the preotic NC results in malformed septal branches, which correspond to the direct contribution of the crest cells, and redundant formation of the coronary orifices without obvious great vessel anomalies. These results suggest that the preotic NC may be more directly involved in coronary artery formation by controlling the integrity of the vascular wall and determining the site of orifices in a manner distinct from those for the postotic NC. Preotic NCCs migrating into the heart appear to differentiate into other cell types in addition to SMCs. Many of these cells distribute mainly in the interventricular septum and papillary muscles in a scattered pattern. Recently, Fukuda and colleagues [26] , [27] have reported the presence of a NC-derived stem cell population in the heart, which can differentiate into various cell types, including cardiomyocytes. By contrast, our present study shows that preotic NCCs do not differentiate into cardiomyocytes, at least in embryonic stages ( Supplementary Fig. S12 ). The comparison between these NC derivatives deserves further study. It is also noteworthy that r4-derived NCCs, which constitute PA2 ectomesenchyme, are the major population of preotic NCCs migrating into the heart and contributing coronary artery formation. PA2 mesoderm-derived cells have been reported to migrate into the heart as the leading edge of the second heart field [28] , [29] . Possible interaction between migratory preotic NCCs and PA2-derived mesodermal cells may also warrant further investigation. We also showed the role of Edn signalling in the remodelling of coronary arteries in mouse and chick embryos. The similarity of the Edn1 -/ Ednra -null phenotype in mouse to the NC ablation in chick suggests that the preotic NC is the target of Edn signalling in coronary remodelling. We have previously reported that Edn1 activates the G-protein-coupled receptor Ednra on preotic NCCs migrating into the first PA, and specifies mandibular identity through G q /G 11 -dependent signalling [18] . This and the present findings indicate that Edn1 activates different signalling and genetic programmes in preotic NCCs in different contexts. Interestingly, coronary artery dilation in the interventricular septum is observed in NC-specific G 12 /G 13 -deficient mice rather than G q /G 11 -deficient mice [30] . Ednra has been reported to couple with G 12 /G 13 as well as G q /G 11 and activate Rho signalling in various cell types, including vascular SMCs [31] , [32] . Rho signalling is a key regulator of various cell behaviours, such as migration, differentiation and remodelling, in vascular SMCs [33] , [34] . Taken together, we speculate that Edn1/Ednra may activate Rho signalling in preotic NCCs through a G 12 /G 13 -dependent pathway to modulate coronary artery remodelling. In the present study, we detected Edn1 expression in cushion endocardium and proximal coronary endothelium, near which Ednra -expressing NCCs were distributed at the critical stage for coronary formation around E12.5–E14.5. This expression pattern suggests the possibility that the Edn signalling may serve as a local cue for the recruitment of preotic NCCs and their differentiation into SMCs in the coronary vasculature. Vascular SMCs originate from different sources depending on the region [11] . In the coronary arteries, SMCs have been proved to be mainly of proepicardial origin [12] , [35] , [36] , [37] . On the other hand, the heterogeneity of coronary artery SMCs has also been suggested by a number of studies, and NCCs and second heart field-derived cells have been considered as candidate sources [15] , [38] , [39] . However, lack of direct evidence has lead many investigators to question the NC contribution to coronary artery SMCs [11] . Our present findings provide direct evidence by identifying the preotic NC as another source. Especially, preotic NCCs preferentially contribute to the septal and conotruncal regions, which appear less accessible to epicardial cells compared with the ventricular free walls. The origin and patterning of the coronary arteries exhibit remarkable diversity among vertebrate species [40] . In fish, the coronary circulation originates from postbranchial vessels corresponding to the dorsal aorta. After lungs replace gills during evolution, the origin gradually shifts from the dorsal aorta to the ventral aorta, which is the closest supply of oxygenated blood to the heart. Such phylogenetic diversity may be associated with differences in migration and interaction of heterogeneous cell populations involving NCCs. Indeed, ablation of the preotic NC affects the number and position of coronary ostia and vascular morphology. Furthermore, the interventricular septum, where preotic NCCs mostly migrate, is a novel structure in vertebrate evolution and is phylogenetically diverse in its morphology and patterns of blood supply [41] , [42] . These findings lead us to speculate that preotic NC may provide species-specific patterning information as observed in craniofacial development [43] , [44] . Heterogeneity of coronary SMCs gives another implication in the pathophysiology of coronary artery disease, a major cause of death throughout the world. Previous studies have suggested that susceptibility to atherosclerosis is highly associated with cell lineage in humans and experimental animals [45] , [46] , [47] . NC-derived SMCs and mesoderm-derived SMCs are shown to be different in growth and agonist-induced gene expression patterns [48] , [49] . A recent report demonstrated that NC-derived SMCs were more prone to calcification than those of mesodermal origin [50] . Taken together with these previous findings, our results may provide a new basis for the understanding of the pathophysiology of coronary artery disease. Animals Edn1 KO ( Edn1 –/– ) mice [21] , Ednra KO ( Ednra EGFP/EGFP , EGFP -knock-in) mice [24] , Wnt1-Cre /R26R reporter mice [15] , [51] and R4::Cre;Z/AP mice [52] , [53] have been described previously. Mutant mice were maintained on a mixed C57BL/6J × ICR background and were housed in an environmentally controlled room at 23±2 °C, with a relative humidity of 50–60% and under a 12-h light:12-h dark cycle. Genotypes were determined by PCR on the tail-tip or amnion DNA using specific primers provided in Supplementary Table S4 . Embryonic ages were determined by timed mating with the day of the plug being E0.5. Fertilized Hojuran chicken ( Gallus gallus ) eggs and Japanese quail ( Cortunix japonica ) eggs were obtained from Shiroyama Keien Farms (Tochigi, Japan) and Motoki Hatchery (Saitama, Japan), respectively, and were incubated in a humidified atmosphere at 37 °C until the embryos reached appropriate stages. All animal experiments were approved by the University of Tokyo and Tokyo Women’s Medical University Animal Care and Use Committee, and were performed in accordance with the institutional guidelines. Ink injection Hearts were collected from mouse and chick embryos at appropriate stages and dipped into heparinized PBS. Then, ink (Kiwa-Guro, Sailor, Japan) was gently injected from the ascending aorta using a glass micropipette. Samples were fixed in 4% paraformaldehyde solution and dehydrated in sequential ethanol solution. To visualize the septal branch, dehydrated samples were immersed in BABB (1:2 benzyl alcohol to benzyl benzoate). Some injected samples were re-dehydrated in ethanol solution and embedded in paraffin. Consecutive section (10 μm) was stained with haematoxylin-eosin stain. β-Galactosidase staining LacZ expression was detected by staining with X-Gal (5-bromo-4-chloro-3-indolyl β- D -galactoside) for β-galactosidase activity. Section staining was performed as described previously [54] . For sections, samples were embedded in optical coherence tomography compound, cryosectioned and subjected to X-gal staining. Some sections were counter stained with haematoxylin (Muto Pure Chemicals, Japan). Z/AP staining Z/AP staining has been described previously [55] . E9.5, E11.5 and E14.5 embryos were fixed in 4% paraformaldehyde and rinsed in PBS. After a fixation, samples were rinsed in NTMT (NaCl 0.1 M, Tris–HCl 0.1 M(pH9.5), MgCl 2 0.05 M and Tween20 (0.1%). Nitroblue tetrazolium (3.5 μl; Roche 1383213) and 5-bromo-4-chloro-3-indolyl phosphate (3.5 μl; Roche 1383221) per ml of NTMT were used for the staining. Hearts were dissected and stained as whole mount or cryostat sections. Immunohistochemistry Embryo cryosections (12–16 μm) were immunostained using the following antibodies: rat monoclonal anti-GFP (Nacalai Tesque, Kyoto, Japan; 1:200), rabbit anti-GFP (Medical and Biological Laboratories, Nagoya, Japan; 1:250), mouse monoclonal anti-quail cell (QCPN; Developmental Studies Hybridoma Bank; 1:30), Rabbit polyclonal anti-β-galactosidase (Rockland; 1:1,000), mouse monoclonal anti-actin α-smooth muscle (1A4; Sigma; 1:1,000), rabbit anti-SM22α (Abcam; 1:200), rat anti-mouse CD31 (BD Pharmingen; 1:100) and mouse anti-desmin (Developmental Studies Hybridoma Bank; 1:100). Signals were visualized with FITC (fluorescein isothiocyanate)- or TRITC-conjugated secondary antibodies specific for the appropriate species. Some sections were treated with biotin-conjugated secondary antibodies and visualized using the VECTASTAIN ABC System (Vector Laboratories), streptavidin-FITC (Dako; 1:200), streptavidin-TRITC (Beckman Coulter; 1:200), or streptavidin-APC (eBioscience; 1:200). Nuclei were visualized with TO-PRO-3 (Molecular Probes). Fluorescent signals were visualized with a computer-assisted confocal microscope (Nikon D-ECLIPSE C1 and EZ-C1 software (Nikon). In situ hybridization In situ hybridization was performed on cryosections (16 μm) using the Edn1 probe as previously described [21] , [24] . Three-dimensional reconstructions Each paraffin-embedded section (4–10 μm) was used for reconstruction. Digital images of the stained sections were loaded into Amira (Visage Imaging, Inc.) with a voxel size appropriate to section thickness. Images were aligned and concerned regions (QCPN-positive signals or the septal branch) were labelled. The labels were resampled to iso-volumetric voxel dimensions, and these smoothed data sets were transformed into a surface by triangulation. The number of triangles was reduced using the SmoothSurface module of Amira. Quail–chick chimera and ablation of the NC Quail–chick chimeras have been described previously [7] , [56] . After an incubation of fertilized quail and chicken eggs in a humid chamber at 37 °C, window was cut through the shell and embryo were visualized with India ink (black ink, Rotring, Germany) diluted 1:10 in saline solution, injected into the subgerminal cavity. Stages of host chicken and donor quail embryos were match as closely as possible. Ablation of the neural folds, including premigratory NC, was performed by manual extirpation using electrolytically sharpened tungsten needles. For premigratory cranial NC (from the midbrain to the r5) of chimera and ablation, the 4- to 7-ss embryos were used. Because of whole staining embryos using HNK1 antibody (data not shown), cranial NCCs of the 8-ss embryos were migrated. For premigratory cardiac NC (from the r6–r8 and somite 4) of chimera and ablation, the 6- to 9-ss embryos were used. Sham-operated embryos were produced by tearing the vitelline membrane with no further surgery. For control embryos the windows were opened and the somite with no treatment were counted. Quail–chick proepicardium chimera Quail–chick proepicardium (PEO) chimeras have been described previously [57] . Stage 16–17 quail hearts were inspected to confirm that the PEO was not attached to the dorsal wall of the heart. Using an eggshell membrane, the quail PEO was isolated together with the sinus venosus and transplanted behind the chick heart. After an appropriate incubation period, the embryos were killed, and their hearts were subjected to immunostaining. In-ovo fluorescent dye injection Method has been described previously [29] , [58] . Fluorescent dye injection was performed on 8-ss chick embryos. Micropipettes were filled with CM-DiI (Molecular Probes) or CFDA/DiO mixture (1:1; Molecular Probes) in ethanol or N,N-dimethylformamide (Wako) was diluted 1:1, or 1:2 in tetraglycol (Sigma) to yield working solutions of 1.0, or 2.5 mg ml −1 , respectively. Pharmacological inactivation of Edn signalling in ovo The method has been described previously [59] . Thirty microlitre olive oil drop was introduced onto the shell membrane at 48 h of incubation. At day 12, embryos were collected. In the bosentan-treated group, bosentan (Actelion, Ltd) was suspended in the oil at the 5 mg ml −1 , whereas only oil was given to the control group. How to cite this article: Arima Y. et al . Preotic neural crest cells contribute to coronary artery smooth muscle involving endothelin signalling. Nat. Commun. 3:1267 doi: 10.1038/ncomms2258 (2012).